Self-assembled conjoined-cages A self-assembled coordination cage usually possesses one well-defined three-dimensional (3D) cavity whereas infinite number of 3D-cavities are crafted in a designer metal-organic framework. Construction of a discrete coordination cage possessing multiple number of 3D-cavities is a challenging task. Here we report the peripheral decoration of a trinuclear [Pd 3 L 6 ] core with one, two and three units of a [Pd 2 L 4 ] entity for the preparation of multi-3D-cavity conjoined-cages of [Pd 4 (L a ) 2 (L b ) 4 ], [Pd 5 (L b ) 4 (L c ) 2 ] and [Pd 6 (L c ) 6 ] formulations, respectively. Formation of the tetranuclear and pentanuclear complexes is attributed to the favorable integrative self-sorting of the participating components. Cage-fusion reactions and ligand-displacement-induced cage-to-cage transformation reactions are carried out using appropriately chosen ligand components and cages prepared in this work. The smaller [Pd 2 L 4 ] cavity selectively binds one unit of NO 3 − , F − , Cl − or Br − while the larger [Pd 3 L 6 ] cavity accommodates up to four DMSO molecules. Designing aspects of our conjoined-cages possess enough potential to inspire construction of exotic molecular architectures. The construction of metal directed self-assembled complexes was pioneered by Lehn, Saalfrank, Sauvage, Fujita, Stang, Cotton, Raymond, Newkome, and others during the formative stages of this modern research area [1] , [2] , [3] , [4] , [5] , [6] , [7] , [8] , [9] . A diverse range of molecular architectures including, but not limited to, a variety of geometrical/topological shapes like macrocycles, cages, catenanes, and knots are known [10] , [11] , [12] , [13] . Self-assembled coordination macrocycles (monocyclic) typically possess one well-defined two-dimensional (2D) cavity whereas the coordination cages (polycyclic) usually possess one well-defined three-dimensional (3D) cavity [1] , [2] , [3] , [4] , [5] , [6] , [7] , [8] , [9] . Researchers have been actively exploring the synthesis of near-planar multi(monocyclic) coordination complexes that possess two or more 2D-cavities and the area is well-reviewed [5] , [14] , [15] , [16] . In contrast, coordination cages comprising two or more 3D-cavities are extremely rare and multi-compartmental in their builds [9] , [17] , [18] , [19] , [20] , [21] , [22] , [23] , [24] . Multi-compartment vesicles can facilitate individual chemical processes in distinct adjacent compartments [25] . Such behaviors are known in bio-systems as exemplified by functioning of regulatory mechanisms in prokaryotes [26] . Thus, the process of developing simpler routes for synthesizing multi-3D-cavity host molecules is a compelling and challenging task. The early examples of multi-3D-cavity coordination cages were reported by Lehn and co-workers [17] . Initially, a specific Cu(I)-based box-shaped cationic [M 6 (L a ) 3 (L b ) 2 ] cage containing a 3D-cavity was prepared using a linear bis-bidentate ligand (L a ) and trigonal planar tris-bidentate ligand (L b ) [27] . Subsequently, the linear ligand L a was modified by adding more binding units on its backbone. The modified L a being tris-bidentate and tetrakis-bidentate in nature, afforded [M 9 (L a ) 3 (L b ) 3 ] and [M 12 (L a ) 3 (L b ) 4 ] cages with two and three 3D-cavities, respectively [17] . The general formula of these cationic cages is [M 3n (L a ) 3 (L b ) n ] where M is Cu(I) or Ag(I), n is 2, 3, or 4 and the number of cavities is “ n – 1”. Schmittel et al. [18] prepared another Cu(I)-based [M 6 (L a ) 3 (L b ) 2 ] cage and then subjected the three bound ligands L a to post-modification using two units of a tripodal linker to obtain one unit of a bound macrobicyclic cyclophane entity. Thus, a [M 6 (cyclophane)(L b ) 2 ] type cationic compound, containing three 3D-cavities was prepared. Hardie and co-workers prepared a Cu(II)-based neutral dumbbell-shaped [M 3 (L a ) 2 (dmf) 3 ] cage where L a represents a tri-anionic tripodal tris-monodentate ligand. Two units of the trinuclear cage were linked using a neutral bis-monodentate linear linker (L b ), to afford a neutral [{M 3 (L a ) 2 (dmf)(H 2 O)} 2 (μ-L b )] architecture that contains identical 3D-cavities [19] . A few years ago, we prepared a Pd(II)-based cationic double-decker [M 3 L 4 ] cage possessing two identical 3D-cavities (Fig. 1a ) [20] . We prepared the [M 3 L 4 ] cage using Pd(NO 3 ) 2 and an “E-shaped” neutral tris-monodentate ligand in 3:4 ratio. Our design enables the creation of tuneable cavities by keeping the donor units of the ligand intact and simply modifying the spacer moieties. A few other [Pd 3 L 4 ] complexes were subsequently reported by the research groups of Clever, Yoshizawa and Crowley [21] , [22] , [23] , by suitably modifying the spacer units in the ligand backbones to realize bigger sized [Pd 3 L 4 ] double-cavities. The Crowley group introduced an additional donor site in the ligand design, creating a tetrakis-monodentate ligand that allowed the formation of a [Pd 4 L 4 ] complex with three 3D-cavities arranged in a linear fashion [23] . The environment of central cavity, by virtue of its position, has to be different from a terminal cavity, however, there are subtle differences in the frameworks of the central versus terminal cavities in the design of Crowley. In short, a few examples of [M n L 4 ] multi-cavity cages (where M is Pd(II), “ n ” is 3 or 4) with “ n − 1” cavities (Fig. 1a ) are known. In contrast to the multiple binding sites of the multi-3D-cavity cages, there exist single-3D-cavity systems capable of accommodating multiple variety of guests in site-specific manner [28] , [29] . It is pertinent to note that a variety of 3D-metal−organic frameworks possessing an infinite number of conjoined-cages in their architectures are known [7] . As described above, only a handful of multi-3D-cavity self-assembled cages are known in literature, where the cavities are usually arranged in a linear fashion in their superstructures and the maximum number of cavities is three. Fig. 1: Cartoon representation of the design approaches for making of self-assembled multi-3D-cavity cages. a linearly conjoined homoleptic cages [20] , [23] and b linearly/laterally conjoined targeted homo- and heteroleptic cages (this work). Full size image The processes of construction of coordination cages are sometime classified under narcissistic and integrative self-sorting [30] , [31] that are comparable to certain biological processes [32] , [33] , [34] . Dynamic behaviors of the coordination cages with respect to post-modifications such as cage-fusion reactions [35] and ligand-displacement-induced cage-to-cage transformations [36] are important studies of current interest. Construction of multi-3D-cavity cages, understanding related self-sorting processes and subjecting the cages to post-modifications are therefore attractive and fundamental aspects of supramolecular coordination chemistry. In the present work, we report a family of rationally designed modular multi-cavity Pd(II)-based coordination cages where 3D-cages of two varieties, namely [Pd 2 L 4 ] and [Pd 3 L 6 ] are conjoined in a linear or lateral manner (Fig. 1b ). We have named such architectures as “self-assembled conjoined - cages”. A family of conjoined 3D-cages of [Pd 4 (L a ) 2 (L b ) 4 ], [Pd 5 (L b ) 4 (L c ) 2 ] and [Pd 6 (L c ) 6 ] formulations containing two, three, and four cavities, respectively, has been prepared (Fig. 1b ). The smaller peripheral cavity of the conjoined-cages selectively binds certain anions while the larger central cavity contains solvent molecules. Dynamic behaviors of the conjoined-cages depicting cage-fusion reactions and ligand-displacement-induced cage-to-cage transformations are studied. Narcissistic and integrative self-sorting processes are demonstrated in connection with the synthesis of the cages. Design and synthesis of the ligands The complexation of Pd(II) with suitable nonchelating bidentate ligands is known to yield [Pd m L 2m ] complexes. The value of “ m ” can be qualitatively related to the angle subtended by the two coordination vectors of the bound ligand. While [Pd 2 L 4 ] complexes are common and have been widely explored [6] , [37] , [38] , [39] , molecules with [Pd 3 L 6 ], [Pd 4 L 8 ], [Pd 5 L 10 ], [Pd 6 L 12 ], [Pd 7 L 14 ], [Pd 8 L 16 ], [Pd 9 L 18 ], [Pd 12 L 24 ], [Pd 30 L 60 ], [Pd 48 L 96 ] architectures possessing a single-3D-cavity are also known [6] , [40] , [41] , [42] . In order to accomplish the multi-3D-cavity targets shown in Fig. 1b , the first step was to identify two nonchelating bidentate ligands; one capable of forming a [Pd 2 L 4 ] and the other a [Pd 3 L 6 ] complex. Mere identification of any two capable ligands is not sufficient, since the backbones of the chosen ligands need to be integrated in such a manner that the hybrid ligands so obtained can sustain [Pd 2 L 4 ] and [Pd 3 L 6 ] entities within the same superstructure. The objectives include the construction of tetra, penta and hexanuclear complexes shown in Fig. 1b . The ligands designed for this purpose are shown in Fig. 2 . The bidentate ligands L2 and L3 yielded [Pd 2 L 4 ] and [Pd 3 L 6 ] architectures, respectively. The builds of L2 and L3 are integrated in the designs of the tri-/tetradentate ligands L5 / L6 . Fig. 2: Structure of the ligands. The ligands L1–L6 . Full size image The ligand L1 was prepared as reported [20] and L2 by a modified method [43] . The new ligands L3 – L6 were synthesized as described hereafter. The ligands L2 and L3 were obtained by condensation of nicotinoyl chloride hydrochloride with 3-pyridylcarbinol and resorcinol, respectively. The ligand L4 was obtained by selective cleavage of one of the ester linkages of L1 , whereas selective condensation of nicotinic acid with resorcinol resulted in the ligand L4′ . The ligand L5 was synthesized by condensation of L4 with L4′ , whereas the ligand L6 was prepared by condensation of L4 with resorcinol. The ligands were characterized by nuclear magnetic resonance (NMR) spectroscopy and electrospray ionization mass spectrometry (ESI-MS) techniques. Ligand L1 upon complexation with Pd(NO 3 ) 2 forms a double-decker architecture [(NO 3 ) 2 ⊂ Pd 3 ( L1 ) 4 ](NO 3 ) 4 , 1a [20] . [Pd 2 L 4 ] entity Complexation of Pd(NO 3 ) 2 with the ligand L2 in 1:2 ratio was carried out in dimethyl sulfoxide (DMSO)- d 6 . Spontaneous assembly of the components resulted in the complex [NO 3 ⊂ Pd 2 ( L2 ) 4 ](NO 3 ) 3 , 2a within 10 min at room temperature (Fig. 3a ). The 1 H NMR spectrum of the solution (Fig. 4a ) contained multiple sets of signals showing complexation induced downfield shift for relevant protons. Multiple sets of signals are typically associated with either the existence of a dynamic equilibrium of two or more complexes [44] of different formulations or a single complex [44] with multiple isomers where the environment around the bound ligand units differs in each isomer. The ligand L2 , being unsymmetrical, can exist in two possible orientations when bridged between two metal centers. Consequently, four isomeric molecular architectures of [Pd 2 L 4 ] composition (diastereomers) differing in the relative orientations of the bound ligand units are possible. While a statistical mixture of diastereomers in 2a was supported by the 1 H NMR spectrum of the sample, the [Pd 2 L 4 ] composition was proposed based on ESI-MS studies. The addition of one equivalent of TBAX (tetra- n -butylammonium salts) (X = F − , Cl − or Br − ) to a solution of 2a resulted in the corresponding anion exchanged products [X ⊂ Pd 2 ( L2 ) 4 ](NO 3 ) 3 , 2b–2d within 5 min at 70 °C (Fig. 3b ), which exhibited downfield shift of pyridine-α protons. The presence of a NO 3 − ion in the cavity and its templating role was further supported by the fact that complexation of Pd(BF 4 ) 2 with the ligand L2 in 1:2 ratio provided a mixture of several unidentified products. This mixture could be converted to [X ⊂ Pd 2 ( L2 ) 4 ](BF 4 ) 3 , 2a′-2d′ (X = NO 3 − , F − , Cl − , and Br − , respectively), by the addition of one equivalent of the corresponding TBAX, within 5 min at 70 °C. The representative complexes 2b and 2a′ were also characterized by ESI-MS studies. The crystal structure of 2c supported the [Pd 2 L 4 ] architecture (Fig. 5a ) with an encapsulated Cl − ion. The two possible orientations for each ligand strand perhaps introduce partial occupancies for –C(O)– and –CH 2 – at both ends of the –C(O)OCH 2 – spacer moiety. The occupancies could not be resolved properly, and the crystal structure represents a mixture of the four isomeric complexes. Fig. 3: Synthetic scheme for the complexes 2a−2d, 3a−6a, and 4e/4f. Self-assembled coordination cages featuring one or more 3D-cavity constructed by complexation of Pd(NO 3 ) 2 with appropriate ligand(s) to afford a/b/c/d/e homoleptic complexes; f/g heteroleptic complexes via integrative self-sorting; k mixture of homoleptic complexes via narcissistic self-sorting. Cage-fusion reactions to yield h/i heteroleptic complexes (however, no fusion in the case of j ). Full size image Fig. 4: Characterization of the complexes 2a−6a and 4e/4f. Partial 1 H NMR spectra (400 MHz, DMSO- d 6 , 300 K) of a cage 2a (diastereomeric mixture), b cage 3a (trinuclear), c mixture of 4e and 4f (tri- and hexanuclear), d cage 4a (tetranuclear), e cage 5a (pentanuclear), and f cage 6a (hexanuclear). Full size image Fig. 5: Crystal structures showing the cationic portions. a Cage 2c (binuclear), b cage 3a (trinuclear), c cage 4acI (tetranuclear), d cage 5c (pentanuclear), and e cage 6c (hexanuclear) (encapsulated guests, counter-anions, solvents, and hydrogen atoms are excluded for clarity. ORTEP diagram for complexes and suitable crystal structures showing encapsulated guests are available in the Supplementary Figs. 134 – 143 ). Full size image [Pd 3 L 6 ] entity The complexation of Pd(NO 3 ) 2 with the ligand L3 in 1:2 ratio was carried out in DMSO- d 6 . Spontaneous assembly of the components resulted in the complex [Pd 3 ( L3 ) 6 ](NO 3 ) 6 , 3a within 10 min at room temperature (Fig. 3c ) and the 1 H NMR spectrum of the solution (Fig. 4b ) showed a single set of signals where a downfield shift was seen in the positions of the pyridine-α protons. The [Pd 3 L 6 ] composition of 3a was proposed based on ESI-MS studies. Synthesis of the complexes [Pd 3 ( L3 ) 6 ](X) 6 , 3b – 3f (for X = BF 4 − , ClO 4 − , OTf − , PF 6 − and SbF 6 − , respectively) was completed within 10 min at room temperature and the 1 H NMR spectra of these complexes are all comparable (except for minor differences in the signal of H g3 ). Thus, the role of anion templation in the formation of these trinuclear complexes ( 3a – 3f ) was ruled out. However, encapsulation of solvent molecules in the cavity of the complexes is likely. ESI-MS study of the representative complex [Pd 3 ( L3 ) 6 ](BF 4 ) 6 , 3b supported the [Pd 3 L 6 ] composition. 1 H NMR spectra of the complex 3a were recorded at various concentrations. At a very low concentration (1 mM with respect to Pd(II)) the complex 3a started dissociating, releasing approximately 19% of uncoordinated ligand L3 . Interestingly, ~7% of L3 existed as a binuclear complex [Pd 2 ( L3 ) 4 ](NO 3 ) 4 , 3g , of the [Pd 2 L 4 ] variety, while the trinuclear 3a remained the major species. At higher concentration, (30 mM with respect to Pd(II)) approximately ~6% of L3 existed as a tetranuclear complex [Pd 4 ( L3 ) 8 ](NO 3 ) 8 , 3h , of the [Pd 4 L 8 ] variety, whereas the trinuclear 3a remained the major species (see Supplementary Fig. 30 ). 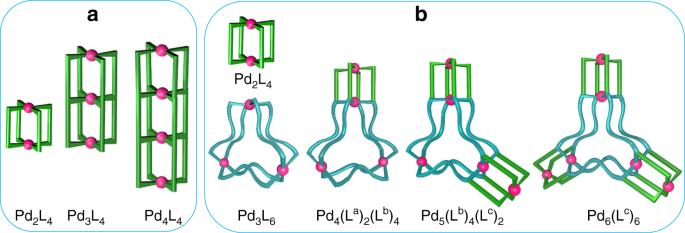Fig. 1: Cartoon representation of the design approaches for making of self-assembled multi-3D-cavity cages. alinearly conjoined homoleptic cages20,23andblinearly/laterally conjoined targeted homo- and heteroleptic cages (this work). The evolution of the smaller 3g and larger sized 3h (Supplementary Discussion 1 and Supplementary Table 1 ) at lower and higher concentrations, respectively, were proposed based on entropic concepts [44] . The formation of 3g and 3h was also confirmed using ESI-MS data (see Supplementary Figs. 31 , 32 ). Attempts to grow single crystals of these complexes proved unsuccessful. PM6 optimized structures of 3g and 3h are given in lieu of the crystal structures (see Supplementary Fig. 132 ). The bidentate ligand L3 possesses a central aromatic spacer and two terminal 3-pyridyl moieties connected by ester linkages. A few ligands of comparable designs with amide linkages are known, which form [Pd 2 L 4 ] complexes [45] , [46] , [47] . The amide linkages are somewhat rigid and are capable of interacting with counter-anions inside the corresponding cavity, when suitably oriented thereby influencing the formation of smaller [Pd 2 L 4 ] complexes. The observed strong preference of L3 towards the formation of a [Pd 3 L 6 ] complex was rather surprising. Probably, the ester linkages are not suitable for anion binding and their flexible nature allows conformational changes when required. In any case, we needed a ligand, which would yield a [Pd 3 L 6 ] architecture, regardless of the counter-anion present, within a reasonable concentration range. The ligand L3 fits this requirement and satisfies few other criteria necessary to achieve the targets (shown in Fig. 1b ). The crystal structure of the complex 3a revealed a bent conformation of the bound ligand moieties, where the donor atoms are present at the convex face of the curved ligand (Fig. 5b ). Four DMSO molecules are located inside the cavity and the counter-anions are present outside. Conjoined - cages and differential binding The next target was a [Pd 4 (L a ) 2 (L b ) 4 ] complex that can be visualized as a linear conjoin of a [Pd 2 L 4 ] cage with a [Pd 3 L 6 ] cage. Therefore, complexation of Pd(NO 3 ) 2 (4 equiv.) with a mixture of the ligands L3 (2 equiv.) and L5 (4 equiv.) was carried out in DMSO- d 6 . Integrative self-sorting of these components required 4 h at room temperature or 1 h at 70 °C, as revealed by monitoring of 1 H NMR spectra, yielding [NO 3 ⊂ Pd 4 ( L3 ) 2 ( L5 ) 4 ](NO 3 ) 7 , 4a (Fig. 3f ). The 1 H NMR spectrum of the solution (Fig. 4d ) showed a single set of peaks where a downfield shift was seen in the positions of the pyridine-α protons. Addition of TBAX (X = F − , Cl − , or Br − ) to a solution of 4a resulted in the corresponding anion exchanged products [X ⊂ Pd 4 ( L3 ) 2 ( L5 ) 4 ](NO 3 ) 7 , 4b–4d (for X = F − , Cl − , and Br − , respectively) within 5 min at 70 °C. Addition of AgCl to a solution of 4a took longer time for the complete anion exchange when carried out at room temperature, however, at an initial stage partial anion exchange was observed (a mixture of 4a and 4c) as confirmed by 1 H NMR study. 1 H NMR spectra of the solution recorded at an intermediate stage revealed the presence of a mixture of 4a and 4c . Such a mixture was used for growing single crystals and crystals were obtained from two of the crystallization conditions. Crystal structures obtained from both the samples displayed partial occupancies of encapsulated NO 3 − /Cl − ion. The crystal structure of 4acI , revealed the formation of a tetranuclear complex where two cavities are linearly conjoined (Fig. 5c ). The smaller cavity accommodated a NO 3 − /Cl − ion (with partial occupancies) and four DMSO molecules were present inside the bigger cavity. The counter-anions and a few solvent molecules were located outside the cavities. The crystal structure of 4acII is provided in the Supplementary Information . As explained earlier, the complexation of Pd(NO 3 ) 2 with ligand L3 yielded the homoleptic complex 3a . It is also relevant to discuss the complexation behavior of Pd(NO 3 ) 2 with ligand L5 . Since the ligand L5 structurally resembles a combination of L2 and L3 , hence the binding sites of L5 are suited for making [Pd 2 L 4 ] and [Pd 3 L 6 ] entities. Therefore, we pondered reasonable architectures where all three donor sites of L5 and all four acceptor sites around Pd(II) are completely utilized and the anticipated [Pd 2 L 4 ] and [Pd 3 L 6 ] like entities are sustained. A structure could not be readily visualized, nevertheless, complexation of Pd(NO 3 ) 2 with ligand L5 in 3:4 ratio was performed in DMSO- d 6 by stirring the mixture for 1 h at 70 °C (Fig. 3d ). 1 H NMR spectrum of the solution (Fig. 4c ) exhibited two sets of signals, which appear downfield relative to the corresponding ligand protons. The 1 H, 13 C, H-HCOSY, and NOESY NMR data along with description about the complexes are given in supplementary section (see Supplementary Figs. 96 – 100 and Supplementary Discussions 2 – 4 ). While the 1 H NMR spectra recorded at different temperatures (30 to 100 °C range) (see Supplementary Fig. 101 ) did not show any noticeable change those recorded at different concentrations (see Supplementary Fig. 102 ) showed changes in the relative intensities of the signals, indicating the coexistence of two well-defined complexes. Their architectures could not be readily predicted. ESI-MS data provided evidence to propose the formation of [NO 3 ⊂ Pd 3 ( L5 ) 4 ](NO 3 ) 5 , 4e and [(NO 3 ) 2 ⊂ Pd 6 ( L5 ) 8 ](NO 3 ) 10 , 4f (see Supplementary Fig. 103 ). The structures of 4e and 4f are such that the L2 -like fragment of L5 got manifested in the [Pd 2 L 4 ] form (in both 4e and 4f ), whereas the L3 -like fragment of L5 evolved in the [Pd 2 L 4 ] (in 4e ) and [Pd 4 L 8 ] (in 4f ) forms (see Supplementary Fig. 95 ). This observation is in line with the fact that the complexation of Pd(NO 3 ) 2 with ligand L3 resulted in very small proportions of [Pd 2 ( L3 ) 4 ](NO 3 ) 4 , 3g and [Pd 4 ( L3 ) 8 ](NO 3 ) 8 , 3h at low and high concentrations, respectively. Addition of AgCl to a mixture of 4e and 4f resulted in the anion exchanged products [Cl ⊂ Pd 3 ( L5 ) 4 ](NO 3 ) 5 , 4g and [(Cl) 2 ⊂ Pd 6 ( L5 ) 8 ](NO 3 ) 10 , 4h within 30 min at room temperature (see Supplementary Fig. 104 ). The compositions of 4g and 4h were also supported by ESI-MS data (see Supplementary Fig. 105 ). Attempts to grow single crystals of these complexes proved unsuccessful. PM6 optimized structures of 4g and 4h are given in lieu of the crystal structures (see Supplementary Fig. 133 ). A [Pd 5 (L b ) 4 (L c ) 2 ] type complex that approximates a lateral conjoining of two [Pd 2 L 4 ] cavities around a [Pd 3 L 6 ] core was our next target. The complexation of Pd(NO 3 ) 2 (5 equiv.) with a mixture of the ligands L5 (4 equiv.) and L6 (2 equiv.) was carried out in DMSO- d 6 in anticipation of the integrative self-sorting behavior of the system (Fig. 3g ). The self-sorting of the components occurred within 4 h at room temperature (or 1 h at 70 °C), as revealed by 1 H NMR study, yielding [(NO 3 ) 2 ⊂ Pd 5 ( L5 ) 4 ( L6 ) 2 ](NO 3 ) 8 , 5a . The 1 H NMR spectrum of the solution (Fig. 4e ) showed a single set of peaks where pyridine-α proton signals appear downfield relative to those of the ligands. The composition of 5a was proposed based on ESI-MS data. Addition of TBAX (X = F, Cl, or Br) to a solution of 5a resulted in the corresponding anion exchanged products [(X) 2 ⊂ Pd 5 ( L5 ) 4 ( L6 ) 2 ](NO 3 ) 8 , 5b – 5d (for X = F − , Cl − , and Br − , respectively) within 5 min at 70 °C. The crystal structure of the complex 5c revealed laterally conjoined cavities as anticipated (Fig. 5d ). The two smaller cavities accommodated a Cl − ion each and four DMSO molecules were present inside the larger cavity. The counter-anions and a few solvent molecules were located outside the cavities. The complexation of Pd(NO 3 ) 2 with the ligand L6 in 1:1 ratio was carried out in DMSO- d 6 (Fig. 3e ). Spontaneous assembly of the components resulted in the complex [(NO 3 ) 3 Pd 6 ( L6 ) 6 ](NO 3 ) 9 , 6a within 1 h at room temperature or 20 min at 70 °C. The 1 H NMR spectrum of the solution (Fig. 4f ) showed a single set of signals where the peaks of pyridine-α protons showed a downfield shift. The [Pd 6 L 6 ] composition of 6a was proposed based on ESI-MS data. Since the ligand L6 structurally resembles a combination of L2 and L3, complexation of Pd(II) with L6 affords the targeted [Pd 6 (L c ) 6 ] complex. Thus, our objective of synthesizing a complex containing three [Pd 2 L 4 ] cavities laterally conjoined with a [Pd 3 L 6 ] core was successfully accomplished. Addition of TBAX (X = F − , Cl − , or Br − ) to a solution of 6a resulted in the corresponding anion exchanged products [(X) 3 ⊂ Pd 6 ( L6 ) 6 ](NO 3 ) 9 , 6b – 6d (for X = F − , Cl − , and Br − , respectively) within 5 min at 70 °C. The composition of 6a and 6c were also supported by ESI-MS data. The crystal structure of the complex 6c revealed laterally conjoined cavities as anticipated (Fig. 5e ). The three smaller cavities accommodated a Cl − ion each and three DMSO molecules were present inside the larger cavity. The counter-anions and a few solvent molecules were located outside the cavities. It was interesting to note that a combination of Pd(BF 4 ) 2 , L3 and L5 in 4:2:4 ratio resulted in a mixture of several unidentified products. The mixture of products could, however, be converted to [X ⊂ Pd 4 ( L3 ) 2 ( L5 ) 4 ](BF 4 ) 7 , 4a′−4d′ (X = NO 3 − , F − , Cl − , and Br − , respectively) by addition of the corresponding TBAX and the process was complete in 1 h at 70 °C. Similarly, a mixture of products was obtained when (i) Pd(BF 4 ) 2 , L5 and L6 were combined in 5:4:2 ratio or (ii) Pd(BF 4 ) 2 and L6 were combined in 1:1 ratio. These mixtures could be converted to discrete (i) [(X) 2 ⊂ Pd 5 ( L5 ) 4 ( L6 ) 2 ](BF 4 ) 8 , 5a′ − 5d′ and (ii) [(X) 3 ⊂ Pd 6 ( L6 ) 6 ](BF 4 ) 9 , 6a′ − 6d′ complexes via the addition of TBAX (X = NO 3 − , F − , Cl − , or Br − ). Cage-fusion reactions Cage-fusion reactions were investigated by combining any two cages, from the pool of 3a , 4a , 5a , 6a , and 4e . Although 4e and 4f coexist, for ease of understanding and calculation, the presence of 4f was neglected. The cage-fusion reactions were monitored by recording 1 H NMR spectra of the solutions as a function of time. The combination of the two homoleptic systems 3a and 4e in 1:3 ratio in DMSO- d 6 resulted in the heteroleptic system 4a within 4 h at room temperature or 20 min at 70 °C (Fig. 3h ). In another instance, the combination of the homoleptic systems 6a and 4e in 1:3 ratio in DMSO- d 6 resulted in the heteroleptic system 5a , within 4 h at 70 °C (no changes occurred at room temperature) as shown in Fig. 3i . The L3 -like fragment might prefer to form a [Pd 3 L 6 ] entity, however, this fragment in the complex 4e exists in the less preferred [Pd 2 L 4 ] form. Consumption of 4e and the formation of 4a or 5a containing the preferred [Pd 3 L 6 ] entity is considered as the driving force of the cage-fusion reactions. However, a mixture of the homoleptic complexes 3a and 6a remained unchanged even after stirring for 24 h at 70 °C (Fig. 3j ). Presumably, the complex 6a is quite stable and requires higher energy for a reshuffle in its architecture. No cage-fusion was observed when the heteroleptic complexes 4a and 5a were allowed to interact with each other. Similarly, no fusion was observed in experiments involving a homoleptic-heteroleptic pair of complexes such as 3a/4a , 3a/5a , 4e/4a , 4e/5a , 6a/4a , and 6a/5a (see Supplementary Methods and Supplementary Figs. 106 – 117 , for all the cage-fusion reactions). The integrative self-sorting phenomenon could be demonstrated in terms of the synthesis of 4a and 5a in separate reactions using Pd(NO 3 ) 2 and appropriate ligands as shown in Fig. 3f, g . These two integrative self-sorted complexes could also be prepared by cage-fusion reactions as discussed above. Thus, a cage-fusion reaction or direct combination of corresponding metal and ligand components yield the same final product, presumably through different routes [30] . An unsuccessful cage-fusion reaction (or no change) belongs in the category of narcissistic self-sorting. One such example of narcissistic self-sorting is observed when Pd(NO 3 ) 2 is mixed with the ligands L3 and L6 in one-pot (Fig. 3k and Supplementary Fig. 110 ), yielding a mixture of the corresponding homoleptic complexes 3a and 6a only. Ligand-displacement-induced cage-to-cage transformations Subsequently, a variety of ligand-displacement-induced cage-to-cage transformations were attempted as shown in Fig. 6 . A chosen cage was mixed with a calculated amount of externally added ligand(s), whereupon the bound ligand(s) are partially or completely displaced by the incoming ligand(s), leading to complete disappearance of the original cage and formation of a different cage. For example, the cage 3a could be transformed to the cage 6a in a cage-to-cage fashion via the interaction of 3a (2 equiv.) with L6 (6 equiv.) whereupon L3 (12 equiv.) and 6a (1 equiv.) were obtained (Fig. 6b ). The list of successful cage-to-cage transformations include the conversion of 3a to 4a , 5a or 6a (Fig. 6a, g, b ); conversion of 4e to 4a or 6a (Fig. 6e, f ); conversion of 4a to 6a (Fig. 6c ); and conversion of 5a to 6a (Fig. 6d ). The cage-to-cage transformations were monitored by recording 1 H NMR spectra of the solutions as a function of time. All these transformations were complete in about 1 h at 70 °C. Fourteen different combinations were tried out of which seven (mentioned above) were successful (see Supplementary Methods and Supplementary Figs. 118 – 131 , for all ligand-displacement reactions). The cages produced are probably more stable than the reactant cages in a qualitative sense. Fig. 6: Ligand-displacement-induced cage-to-cage transformations. Initial-cage/ligand-input/final-cage/displaced-ligand a system 3a / L5 / 4a / L3 ; b system 3a / L6 / 6a / L3 ; c system 4a / L6 / 6a / L3 & L5 ; d system 5a / L6 / 6a / L5 ; e system 4e / L3 / 4a / L5 ; f system 4e / L6 / 6a / L5 ; g system 3a / L5 & L6 / 5a / L3 (stoichiometry are provided in the figure. The complex 4e coexists with 4f ). Full size image This article demonstrated the construction of multi-3D-cavity coordination cages via decoration of a [Pd 3 L 6 ] core with one or more [Pd 2 L 4 ] units in a linear or lateral fashion, respectively. The metal component used for the preparation of the cages was Pd(NO 3 ) 2 and the cages formed ( 2a , 4a , 5a , and 6a ) were found to encapsulate NO 3 − in their [Pd 2 L 4 ] moieties. The encapsulated NO 3 − could be replaced by halides like F − , Cl − , or Br − by using corresponding TBAX. Notably, AgCl could be also used as a source of Cl − ion. In fact, Clever and co-workers [48] used sparingly soluble AgCl as a source of Cl − that displaced bound BF 4 − ion from the cavity of certain coordination cages, resulting in consumption of AgCl and retention of the more soluble AgBF 4 in solution. We have also demonstrated the use of AgCl where the Cl − ion displaced bound NO 3 − ion from the cavity of some coordination cages whereupon the more soluble AgNO 3 remained in solution [49] . The requirement of the encapsulated anions in the creation of these assemblies was realized when attempts toward synthesizing Pd 2 L 4, [Pd 4 (L a ) 2 (L b ) 4 ], [Pd 5 (L b ) 4 (L c ) 2 ], and [Pd 6 (L c ) 6 ] cages using Pd(BF 4 ) 2 failed and the experiments led to the formation of a mixture of unidentified products. Probably, the formation of the [Pd 2 L 4 ] entity was hindered, due to repulsion between the closely placed metal ions, in the absence of an appropriate anionic template. This hindrance in turn prevented the building of the targeted conjoined-cages. The BF 4 − ion was found to be un-suitable as a template here. The addition of TBAX (where X = NO 3 − , F − , Cl − , and Br − , respectively) to these mixtures yielded the desired cages. Hence, the formation of Pd 2 L 4 , [Pd 4 (L a ) 2 (L b ) 4 ], [Pd 5 (L b ) 4 (L c ) 2 ], and [Pd 6 (L c ) 6 ] cages is feasible only when the smaller cavity is occupied by NO 3 − , F − , Cl − , or Br − , irrespective of the counter-anion present outside the cavity/cavities. Although the formation of the larger cavity (i.e., [Pd 3 L 6 ] entity) is anion independent, this did not help in the formation of corresponding conjoined-cages ( 4a , 5a , and 6a ) since the formation of [Pd 2 L 4 ] entity is essential. Synthesis of the heteroleptic complex 4a through the combination of Pd(NO 3 ) 2 , L3 and L5 in a single-pot is a perfect example of integrative self-sorting behavior [30] , [31] since the homoleptic complexes formed by L3 and L5 were not observed in the final product profile. Integrative self-sorting was also observed for synthesis of the heteroleptic complex 5a from its components, i.e., Pd(NO 3 ) 2 , L5 and L6 . The formation of these heteroleptic complex is probably driven by the propensity of the L3 -like fragment present in L5 (and L6 ) to form [Pd 3 L 6 ]-like entities. The cages 4a and 5a are hitherto unknown examples of heteroleptic complexes wherein ligands of different denticity are coordinated to Pd(II) [8] . Thus, the present set of cages are unique due to their structural features and associated binding properties. The concept of making conjoined-cages, in an effortless manner opens a plethora of possibilities where suitable ligand design can help construct hitherto unknown architectures with unique structures. General The deuterated solvent DMSO- d 6 was obtained from Sigma-Aldrich. NMR spectra were recorded in DMSO- d 6 at room temperature (r.t.) on Bruker AV400 and AV500 spectrometers at 400 and 500 MHz for 1 H NMR, COSY, NOESY and at 100 and 125 MHz for 13 C NMR. Chemical shifts are reported in parts per million (ppm) relative to residual solvent protons (2.50 ppm for DMSO- d 6 in 1 H NMR and 39.50 in 13 C NMR). The ESI mass spectra were recorded on Agilent Q-TOF spectrometers. Single crystal X-ray diffraction analysis was carried out using a Bruker D8 VENTURE instrument. The ligand L1 was synthesized as reported previously [20] . Synthesis and characterization of the ligands Triethylamine (0.24 mL, 1.685 mmol) was added in a dropwise manner to a stirred suspension of nicotinoyl chloride hydrochloride (0.300 g, 1.685 mmol) and 3-pyridylcarbinol (0.184 g, 0.16 mL, 1.685 mmol) in dry dichloromethane (DCM) (30 mL) maintained at 0–5 °C. The mixture was stirred at room temperature for 24 h under nitrogen atmosphere. In order to neutralize the acid, NaHCO 3 solution (10% w/v ) was added slowly to the mixture until the evolution of CO 2 has ceased. The organic layer was washed with distilled water, separated and dried over anhydrous sodium sulfate. Purification of the crude product by column chromatography (ethyl acetate:hexane, 4:6) yielded the ligand L2 as a colorless liquid (0.288 g, yield 80%) (see Supplementary Figs. 1 – 6 ). TLC (ethyl acetate:hexane, 40:60 v/v): R f = 0.4; 1 H NMR (500 MHz, DMSO- d 6 , room temperature): δ 9.12 (d, J = 1.3 Hz, 1H, H f2 ), 8.82 (dd, J 1 = 4.8 Hz, J 2 = 1.6 Hz, 1H, H i2 ), 8.72 (d, J = 1.4 Hz, 1H, H a2 ), 8.57 (m, 1H, H b2 ), 8.32 (m, 1H, H g2 ), 7.93 (d, J = 7.8 Hz, 1H, H d2 ), 7.57 (m, 1H, H h2 ), 7.43 (m, 1H, H c2 ), 5.43 (s, 2H, H e2 ); 13 C NMR (125 MHz, DMSO- d 6 , room temperature): δ 164.6, 153.8, 150.1, 149.5, 149.4, 137.0, 136.1, 131.5, 125.4, 124.0, 123.7, 64.3; HRMS (ESI, CH 2 Cl 2 /CH 3 OH): m/z Calcd. for C 12 H 10 N 2 O 2 : 214.2200, found 215.0820 [M + H] + . Triethylamine (1.02 mL, 7.246 mmol) was added in a dropwise manner to a stirred suspension of nicotinoyl chloride hydrochloride (1.290 g, 7.246 mmol) and resorcinol (0.400 g, 3.633 mmol) in dry DCM (50 mL) maintained at 0–5 °C. The mixture was stirred at room temperature for 24 h under nitrogen atmosphere. In order to neutralize the acid, NaHCO 3 solution (10% w/v ) was added slowly to the mixture until the evolution of CO 2 has ceased. The organic layer was washed with distilled water, separated and dried over anhydrous sodium sulfate. Complete evaporation of the solvent yielded the ligand L3 as an off-white solid (0.872 g, yield 75%) (see Supplementary Figs. 18 – 22 ). Melting point: 235 °C; 1 H NMR (500 MHz, DMSO- d 6 , room temperature): δ 9.28 (m, 2H, H a3 ), 8.91 (m, 2H, H b3 ), 8.48 (m, 2H, H d3 ), 7.66 (m, 2H, H c3 ), 7.60 (t, J = 8.3 Hz, 1H, H f3 ), 7.43 (t, J = 2.3 Hz, 1H,H g3 ), 7.34 (m, 2H, H e3 ); 13 C NMR (125 MHz, DMSO- d 6 , room temperature): δ 163.4, 154.3, 150.8, 150.5, 137.5, 130.2, 125.0, 124.1, 119.9, 116.2; HRMS (ESI, CH 2 Cl 2 /CH 3 OH): m/z Calcd. for C 18 H 12 N 2 O 4 : 320.2989, Found 321.0680 [M + H] + . The ligand, L1 (0.500 g, 1.431 mmol) was dissolved in 35 mL of THF:H 2 O (1:1) to obtain a clear solution. To this 1 mL of 2 N KOH was added and stirred at room temperature for 2 min, followed by addition of 0.5 mL of 4 N HCl. The reaction mixture was dried under vacuo yielding a solid (0.358 g, 97%), which was further purified by column chromatography using DCM:MeOH (3:7) to obtain the ligand L4 . (see Supplementary Figs. 33 – 38 ). Melting point: 223 °C; TLC (DCM:MeOH, 97:3 v/v): R f = 0.3; 1 H NMR (500 MHz, DMSO- d 6 , room temperature): δ 9.31 (s, 1H, H f /H h ), 9.28 (s, 1H, H f /H h ), 8.75 (m, 1H, H a ), 8.65 (m, 1H, H g ), 8.60 (m, 1H, H b ), 7.98 (m, 1H, H d ), 7.48 (m, 1H, H c ), 5.46 (s, 2H, H e ); 13 C NMR (125 MHz, DMSO- d 6 , room temperature): δ 165.3, 163.9, 154.0, 153.4, 149.4, 149.3, 137.3, 136.4, 131.4, 126.8, 125.5, 123.8, 64.7; HRMS (ESI, CH 2 Cl 2 /CH 3 OH): m/z Calcd. for C 13 H 10 N 2 O 4 : 258.2295, Found 259.0722 [M + H] + . To a suspension of nicotinic acid (0.500 g, 4.065 mmol) and resorcinol (0.112 g, 1.018 mmol) in 50 mL dry DCM maintained at 0–5 °C, dimethylaminopyridine (DMAP) (0.062 g, 0.507 mmol) was added followed by N -ethyl- N ´-(3-dimethylaminopropyl)carbodiimide hydrochloride (EDC.HCl) (0.195 g, 1.017 mmol). The reaction mixture was stirred for 12 h under nitrogen atmosphere. In order to neutralize the acid, NaHCO 3 solution (10% w/v ) was added slowly to the mixture until the evolution of CO 2 has ceased. The organic layer was washed with distilled water, separated and dried over anhydrous sodium sulfate. On standing the product precipitated out. It was isolated by filtration and dried under vacuo to obtain the ligand L4 ′ as a pale pink powder. (0.150 g, 68%) (see Supplementary Figs. 39 – 43 ). 1 H NMR (500 MHz, DMSO- d 6 , room temperature): δ 9.80 (d, J = 7.5 Hz, 1H, –OH), 9.24 (m, 1H, H a ), 8.89 (m, 1H, H b ), 8.44 (m, 1H, H d ), 7.64 (m, 1H, H c ), 7.25 (m, 1H), 6.71 (dd, J 1 = 8.2 Hz, J 2 = 2.0 Hz, 3H); 13 C NMR (125 MHz, DMSO- d 6 , room temperature): δ 163.5, 158.4, 154.2, 151.2 150.5, 137.5, 130.0, 125.2, 124.1, 113.3, 112.2, 109.1. To a suspension of 5-((pyridine-3-ylmethoxy)carbonyl)nicotinic acid, L4 (0.250 g, 0.968 mmol) and 3-hydroxyphenyl nicotinate, L4′ (0.208 g, 0.968 mmol) in 15 mL dry dimethylformamide (DMF) maintained at 0–5 °C, DMAP (0.059 g, 0.484 mmol) was added followed by addition of EDC · HCl (0.186 g, 0.968 mmol). The reaction mixture was stirred for 24 h under nitrogen atmosphere. Addition of water to the reaction mixture resulted in the precipitation of product. The product was isolated by filtration and dried under vacuo to obtain the ligand L5 as an off-white solid powder (0.287 g, 65%). (see Supplementary Figs. 44 – 49 ). Melting point: 238 °C; 1 H NMR (500 MHz, DMSO- d 6 , room temperature): δ 9.48 (d, J = 2.1 Hz, 1H, H f5 /H h5 ), 9.41 (d, J = 2.0 Hz, 1H, H f5 /H h5 ), 9.27 (d, J = 1.4 Hz, 1H, H m5 ), 8.91 (m, 1H, H p5 ), 8.83 (s, 1H, H g5 ), 8.75 (s, 1H, H a5 ), 8.58 (m, 1H, H b5 ), 8.49 (m, 1H, H n5 ), 7.88 (m, 1H, H d5 ), 7.67 (m, 1H, H o5 ), 7.61 (t, J = 8.2 Hz, 1H), 7.45 (m, 2H), 7.36 (m, 2H), 5.49 (s, 2H, H e5 ); 13 C NMR (125 MHz, DMSO- d 6 , room temperature): δ 163.7, 163.4, 162.6, 154.3, 154.2, 150.8, 150.7, 150.6, 149.5, 149.5, 137.7, 137.5, 136.2, 131.3, 130.2, 125.7, 125.3, 124.9, 124.1, 123.7, 120.0, 119.8, 116.1, 64.8; HRMS (ESI, DCM:MeOH): m/z Calcd. for C 25 H 17 N 3 O 6 : 455.4190, Found 456.1196 [M + H] + . To a suspension of 5-((pyridine-3-ylmethoxy)carbonyl)nicotinic acid, L4 (0.469 g, 1.816 mmol) and resorcinol (0.100 g, 0.908 mmol) in 15 mL dry DMF maintained at 0–5 °C, DMAP (0.055 g, 0.4541 mmol) was added followed by EDC · HCl (0.348 g, 1.816 mmol). The reaction mixture was stirred for 24 h under nitrogen atmosphere. 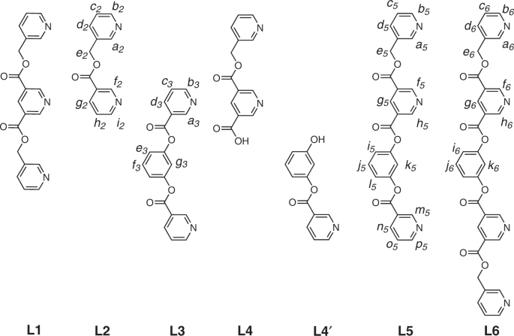Fig. 2: Structure of the ligands. The ligandsL1–L6. Addition of water to the reaction mixture resulted in the precipitation of product. The product was isolated by filtration and dried under vacuo to obtain the ligand L6 as an off-white solid. (see Supplementary Figs. 63 – 68 ). Melting point: 251 °C; 1 H NMR (500 MHz, DMSO- d 6 , room temperature): δ 9.49 (s, 2H, H f6 / H h6 ), 9.42 (s, 2H, H h6 /H f6 ), 8.83 (s, 2H, H g6 ), 8.75 (s, 2H, H a6 ), 8.58 (m, 2H, H b6 ), 7.97 (m, 2H, H d6 ), 7.62 (t, J = 8.3 Hz, 3H, H j6 ), 7.46 (m, 2H, H c6 , H k6 ), 7.37 (m, 2H, H i6 ), 5.49 (s, 4H, H e6 ); 13 C NMR (125 MHz, DMSO- d 6 , room temperature): δ 163.7, 162.6, 154.2, 150.6, 149.6, 149.5, 137.7, 136.2, 131.3, 130.3, 125.7, 125.3, 123.7, 123.7, 120.0, 116.1, 64.8; HRMS (ESI, DCM:MeOH): m/z Calcd. for C 32 H 22 N 4 O 8 : 590.5391, Found 591.1501 [M + H] + . Synthesis and characterization of the complexes The ligand L2 (12.85 mg, 0.059 mmol) was added to a solution of Pd(NO 3 ) 2 (6.91 mg, 0.029 mmol) in 3 mL of DMSO. The reaction mixture was stirred at room temperature for 10 min subsequent, addition of 10 mL of ethyl acetate to the reaction mixture precipitated a white solid, which was separated by centrifugation. The solid was washed with 2 × 2 mL of acetone and dried under vacuum to obtain the complex [NO 3 ⊂ Pd 2 (L2) 4 ](NO 3 ) 3 , 2a as a mixture of diastereomers (16.80 mg, isolated yield 85%) (see Supplementary Figs. 7 – 13 ). Melting point: 232 °C (decomposed); 1 H NMR (500 MHz, DMSO- d 6 , room temperature): δ 9.12 (1H, H f2 ), 8.82 (1H, H i2 ), 8.72 (1H, H a2 ), 8.57 (1H, H b2 ), 8.33 (1H, H g2 ), 7.94 (1H, H d2 ), 7.57 (1H, H h2 ), 7.44 (1H, H c2 ), 5.43 (1H, H e2 ) [multiplicity has not been given as it is a mixture of isomers]; 13 C NMR (125 MHz, DMSO- d 6 , room temperature): δ 162.3, 155.0, 153.2, 153.1, 150.6, 149.3, 149.2, 141.9, 139.3, 139.23, 134.9, 128.7, 128.6, 127.6, 126.4, 118.0, 64.7. DOSY NMR (500 MHz, DMSO- d 6 , 298 K): D = 1.12 × 10 −10 m 2 s −1 ; HRMS (ESI, DMSO): m/z Calcd. for [ 2a –1•NO 3 ] 1+ 1256.0705, found 1256.0688; Calcd. for [ 2a –2•NO 3 ] 2+ 597.0416, found 597.0410; Calcd. for [ 2a –3•NO 3 ] 3+ 377.3651, found 377.3639. Addition of appropriate TBAX to the complex 2a , afforded the complexes [X ⊂ Pd 2 (L2) 4 ](NO 3 ) 3 , 2b–2d . (see Supplementary Methods and Supplementary Figs. 14 , 15 ). A solution of Pd(BF 4 ) 2 was prepared in 0.4 mL of DMSO- d 6 by stirring a mixture of PdI 2 (1.80 mg, 0.005 mmol) and AgBF 4 (1.95 mg, 0.010 mmol) at 90 °C for 30 min The precipitated AgI was separated by centrifugation. The ligand L2 (2.14 mg, 0.010 mmol) was added to the supernatant and the reaction mixture was stirred at 70 °C for 2 h. To this solution tetra- n -butylammonium nitrate (0.76 mg, 0.0026 mmol) was added and heated for 5 min at 70 °C, resulting in the complex [NO 3 ⊂ Pd 2 (L2) 4 ](BF 4 ) 4 , 2a′ . The 1 H NMR spectrum of the complex 2a′ is closely comparable with that of complex 2a . HRMS (ESI, DMSO): m/z Calcd. for [ 2a′ –1•BF 4 ] 1+ 1305.1025, found 1305.0914; Calcd. 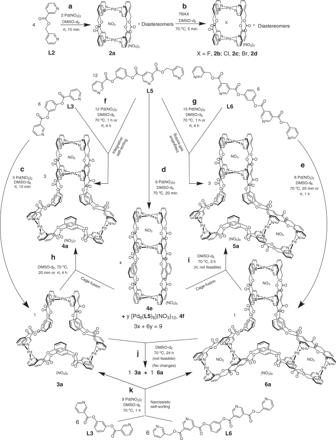Fig. 3: Synthetic scheme for the complexes 2a−2d, 3a−6a, and 4e/4f. Self-assembled coordination cages featuring one or more 3D-cavity constructed by complexation of Pd(NO3)2with appropriate ligand(s) to afforda/b/c/d/ehomoleptic complexes;f/gheteroleptic complexes via integrative self-sorting;kmixture of homoleptic complexes via narcissistic self-sorting. Cage-fusion reactions to yieldh/iheteroleptic complexes (however, no fusion in the case ofj). for [ 2a′ –2•BF 4 ] 2+ 609.5496, found 609.5459; Calcd. for [ 2a′ –3•BF 4 ] 3+ 377.3651, found 377.3636. Complexes [X ⊂ Pd 2 (L2) 4 ](NO 3 ) 3 , 2b′−2d′ were prepared in a similar way. (see Supplementary Methods and Supplementary Figs. 16 , 17 ). The ligand L3 (19.21 mg, 0.059 mmol) was added to a solution of Pd(NO 3 ) 2 (6.91 mg, 0.029 mmol) in 3 mL of DMSO. The reaction mixture was stirred at room temperature for 10 min. Subsequent, slow diffusion of toluene vapor into reaction mixture precipitated a crystalline solid, which was separated by filtration. The solid was dried under vacuum to yield the complex [Pd 3 (L3) 6 ](NO 3 ) 6 , 3a (22.72 mg, isolated yield 58%) (see Supplementary Figs. 23 – 27 ). Melting point: 258 °C (decomposed); 1 H NMR (500 MHz, DMSO- d 6 , room temperature): δ 10.24 (bs, 2H, H a3 ), 9.68 (bs, 2H, H b3 ), 8.65 (bs, 2H, H d3 ), 7.98 (m, 2H, H c3 ), 7.67 (t, J = 8.15 Hz, 1H, H f3 ), 7.37 (m, J = 2.3 Hz, 3H, H e3 /H g3 ); 13 C NMR (125 MHz, DMSO- d 6 , room temperature): δ 161.7, 154.9, 152.6, 150.7, 141.6, 130.7, 128.6, 127.7, 120.6, 116.8; DOSY NMR (500 MHz, DMSO- d 6 , 298 K): D = 9.54 × 10 −11 m 2 s −1 ; HRMS (ESI, DMSO): m/z Calcd. for [ 3a –2•NO 3 ] 2+ 1244.0733, found 1244.0722; Calcd. for [ 3a –5•NO 3 ] 5+ 460.4369, found 460.4373. A solution of Pd(BF 4 ) 2 was prepared in 0.5 mL of DMSO- d 6 by stirring a mixture of PdI 2 (1.80 mg, 0.005 mmol) and AgBF 4 (1.95 mg, 0.010 mmol) at 90 °C for 30 min The precipitated AgI was separated by centrifugation. The ligand L3 (3.20 mg, 0.010 mmol) was added to the supernatant and the reaction mixture was stirred at room temperature for 10 min to afford the complex [Pd 3 (L3) 6 ](BF 4 ) 6 , 3b . The 1 H NMR spectrum of the complex 3b is closely comparable with that of complex 3a except for H g3 , 7.30 (s, 1H, H g3 ). (see Supplementary Fig. 29 ). HRMS (ESI, DMSO): m/z Calcd. for [ 3b –3•BF 4 ] 3+ 833.7355, found 833.7359; Calcd. for [ 3b –4•BF 4 ] 4+ 603.5511, found 603.5510; Calcd. for [ 3b –5•BF 4 ] 5+ 465.4402, found 465.4403. Complexes [Pd 3 (L3) 6 ](X) 6 , 3c – 3f were prepared in a similar way. (see Supplementary Methods and Supplementary Fig. 28 ). The ligands L3 (8.00 mg, 0.025 mmol) and L5 (22.77 mg, 0.050 mmol) were added to a solution of Pd(NO 3 ) 2 (11.52 mg, 0.050 mmol) in 5 mL of DMSO. The reaction mixture was stirred at 70 °C for 1 h to obtain a clear solution. Subsequent, slow diffusion of toluene vapor to the resulting solution precipitated a crystalline solid, which was separated by filtration. The solid was dried under vacuum to obtain the complex [NO 3 ⊂ Pd 4 (L3) 2 (L5) 4 ](NO 3 ) 7 , 4a (18.98 mg, isolated yield 45%). (see Supplementary Figs. 50 – 58 ). Melting point: 260 °C (decomposed); 1 H NMR (500 MHz, DMSO- d 6 , room temperature): δ 11.02 (s, 4H, H f5 ), 10.65 (s, 4H,H h5 ), 10.25 (d, J = 3.5 Hz, 8H, H m5 , H a3 ), 10.05 (s, 4H, H a5 ), 9.66 (d, J = 4.2 Hz, 8H, H p5 , H b3 ), 9.35 (d, J = 4.5 Hz, 4H, H b5 ), 8.92 (s, 4H, H g5 ), 8.66 (d, J = 6.5 Hz, 8H, H n5 , H d3 ), 8.16 (m, 4H, H d5 ), 8.00–7.97 (m, 8H, H o5 , H c3 ), 7.82 (m, 4H, H c5 ), 7.70–7.66 (m, 4H), 7.41–7.35 (m, 16H), 5.56 (m, 8H, H e5 ); 13 C NMR (125 MHz, DMSO- d 6 , room temperature): δ 161.9, 161.8, 161.3, 156.6, 155.0, 152.6, 150.8, 150.8, 149.4, 141.6, 139.5, 134.8, 130.8, 129.1, 129.0, 128.7, 128.6, 127.8, 126.7, 120.9, 120.7, 117.0, 65.3; DOSY NMR (500 MHz, DMSO- d 6 , 298 K): D = 8.51 × 10 −11 m 2 s −1 ; HRMS (ESI, DMSO): m/z Calcd. for [ 4a –3•NO 3 ] 3+ 1065.7228, found 1065.7184; Calcd. for [ 4a –6•NO 3 ] 6+ 501.8678, found 501.8661. Addition of appropriate TBAX to the complex 4a , afforded the complexes X ⊂ Pd 4 (L1) 2 (L2) 4 ](NO 3 ) 7 , 4b – 4d . (see Supplementary Methods and Supplementary Figs. 59 , 60 , 61 ). A solution of Pd(BF 4 ) 2 was prepared in 0.4 mL of DMSO- d 6 by stirring a mixture of PdI 2 (1.80 mg, 0.005 mmol) and AgBF 4 (1.95 mg, 0.010 mmol) at 90 °C for 30 min The precipitated AgI was separated by centrifugation. The ligands L3 (0.80 mg, 0.003 mmol) and L5 (2.28 mg, 0.005 mmol) were added the supernatant and heated at 70 °C for 2 h, yielding an oligomer. To the solution containing the oligomer, tetra- n -butylammonium nitrate (0.38 mg, 0.0012 mmol) in 0.1 mL of DMSO- d 6 was added and heated at 70 °C for 1 h resulting in the formation of complex [NO 3 ⊂ Pd 4 (L3) 2 (L5) 4 ](BF 4 ) 7 , 4a′ . The 1 H NMR spectrum of the complex 4a′ is closely comparable with the data of complex 4a . Complexes [X ⊂ Pd 4 (L3) 2 (L5) 4 ](BF 4 ) 7 , 4b′−4d′ were prepared in a similar way. (see Supplementary Methods and Supplementary Fig. 62 ). The ligands L5 (18.22 mg, 0.040 mmol) and L6 (11.81 mg, 0.020 mmol) were added to a solution of Pd(NO 3 ) 2 (11.52 mg, 0.050 mmol) in 5 mL of DMSO. The reaction mixture was stirred at 70 °C temperature for 2 h. Subsequently, slow diffusion of toluene vapor to the reaction mixture precipitated a crystalline solid, which was separated by filtration. The solid was dried under vacuum to obtain the complex [(NO 3 ) 2 ⊂ Pd 5 (L5) 4 (L6) 2 ](NO 3 ) 8 , 5a (15.76 mg, isolated yield 38%). (see Supplementary Figs. 69 – 77 ). Melting point: 272 °C (decomposed); 1 H NMR (500 MHz, DMSO- d 6 , room temperature): δ 11.04 (s, 8H, H f5 , H f6 ), 10.67 (s, 8H, H h5 , H h6 ), 10.26 (d, 4H, H m5 ), 10.06 (s, 8H, H a5 , H a6 ), 9.68 (s, 4H, H p5 ), 9.36 (d, 8H, H b5 , H b6 ), 8.94 (s, 8H, H g5 , H g6 ), 8.67 (d, J = 8.2 Hz, 4H, H n5 ), 8.18 (bs, 8H, H d5 , H d6 ), 8.01–7.98 (m, 4H, H o5 ), 7.85–7.82 (m, 8H, H c5 , H c6 ), 7.75–7.71 (m, 4H), 7.48–7.41 (m, 16H), 5.64-5.53 (m, 16H, H e5 , H e5 ); 13 C NMR (125 MHz, DMSO- d 6 , room temperature): δ 161.8, 161.3, 156.5, 150.8, 149.3, 141.5, 139.5, 134.8, 130.8, 128.9, 128.6, 126.6, 120.9, 116.8, 65.2; DOSY NMR (500 MHz, DMSO- d 6 , 298 K): D = 5.75 × 10 −11 m 2 s −1 ; HRMS (ESI, DMSO): m/z Calcd. for [ 5a –3•NO 3 ] 3+ 1322.7259, found 1322.7248; Calcd. for [ 5a –4•NO 3 ] 4+ 976.5475, found 976.5474. Addition of appropriate TBAX to the complex 5a , provided the complexes [(X) 2 ⊂ Pd 5 (L5) 4 (L6) 2 ](NO 3 ) 8 , 5b – 5d . (see Supplementary Methods and Supplementary Figs. 78 – 81 ). A solution of Pd(BF 4 ) 2 was prepared in 0.4 mL of DMSO- d 6 by stirring a mixture of PdI 2 (1.80 mg, 0.005 mmol) and AgBF 4 (1.95 mg, 0.010 mmol) at 90 °C for 30 min The precipitated AgI was separated by centrifugation. The ligands L5 (1.82 mg, 0.004 mmol) and L6 (1.18 mg, 0.002 mmol) were added to the supernatant and heated at 70 °C for 2 h to obtain the oligomer. To the solution containing the oligomer, a solution of tetra- n -butylammonium nitrate (0.61 mg, 0.002 mmol) in 0.1 mL of DMSO- d 6 was added and heated at 70 °C for 1 h resulting in the complex [(NO 3 ) 2 ⊂ Pd 5 (L5) 2 (L6) 4 ](NO 3 ) 8 , 5a′ . The 1 H NMR spectrum of the complex 5a′ is closely comparable with the data of complex 5a . Complexes [(X) 2 ⊂ Pd 5 (L5) 2 (L6) 4 ](NO 3 ) 8 , 5a′−5d′ were prepared in a similar way. (see Supplementary Methods and Supplementary Fig. 82 ). The ligand L6 (29.53 mg, 0.050 mmol) was added to a solution of Pd(NO 3 ) 2 (11.52 mg, 0.050 mmol) in 5 mL of DMSO. The reaction mixture was stirred at 70 °C for 20 min to obtain a clear solution. Subsequently, addition of 15 mL of ethyl acetate to the reaction mixture precipitated a white solid, which was separated by centrifugation. The solid was washed with 3 × 3 mL of acetone and dried under vacuum to obtain the complex [(NO 3 ) 3 ⊂ Pd 6 (L6) 6 ](NO 3 ) 9 , 6a (36.98 mg, isolated yield 90%). (see Supplementary Figs. 83 – 88 ). Melting point: 288 °C (decomposed); 1 H NMR: 11.04 (s, 12H, H f6 ), 10.68 (s, 12H, H h6 ), 10.06 (s, 12H, H a6 ), 9.37 (d, J = 8.2 Hz, 12H, H b6 ), 8.94 (s, 12H, H g6 ), 8.19 (d, J = 7.2 Hz, 12H, H d6 ), 7.80 (s, 12H, H c6 ), 7.75 (bs, 6H), 7.48 (bs, 18H), 5.58 (bs, 24H, H e5 ); HRMS (ESI, DMSO): m/z Calcd. for [ 6a –5•NO 3 ] 5+ 923.0424, found 923.0411. Addition of appropriate TBAX to the complex 6a , resulted in the complexes [(X) 3 ⊂ Pd 6 (L6) 6 ](NO 3 ) 9 , 6b–6d . (see Supplementary Methods and Supplementary Figs. 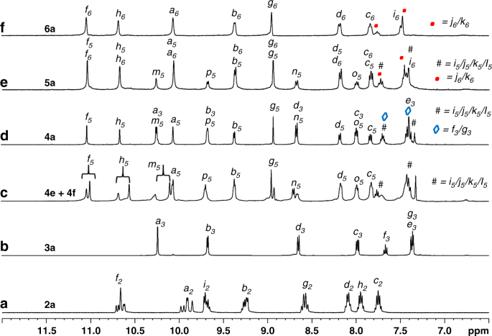Fig. 4: Characterization of the complexes 2a−6a and 4e/4f. Partial1H NMR spectra (400 MHz, DMSO-d6, 300 K) ofacage2a(diastereomeric mixture),bcage3a(trinuclear),cmixture of4eand4f(tri- and hexanuclear),dcage4a(tetranuclear),ecage5a(pentanuclear), andfcage6a(hexanuclear). 89 – 93 ). A solution of Pd(BF 4 ) 2 in 0.4 mL of DMSO- d 6 was prepared by stirring a mixture of PdI 2 (1.80 mg, 0.005 mmol) and AgBF 4 (1.95 mg, 0.010 mmol) at 90 °C for 30 min The precipitated AgI was separated by centrifugation. The ligand L6 (2.95 mg, 0.005 mmol) was added to the supernatant and heated at 70 °C for 2 h to obtain the oligomer. 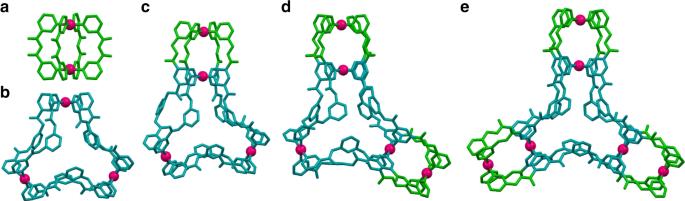Fig. 5: Crystal structures showing the cationic portions. aCage2c(binuclear),bcage3a(trinuclear),ccage4acI(tetranuclear),dcage5c(pentanuclear), andecage6c(hexanuclear) (encapsulated guests, counter-anions, solvents, and hydrogen atoms are excluded for clarity.ORTEPdiagram for complexes and suitable crystal structures showing encapsulated guests are available in the Supplementary Figs.134–143). 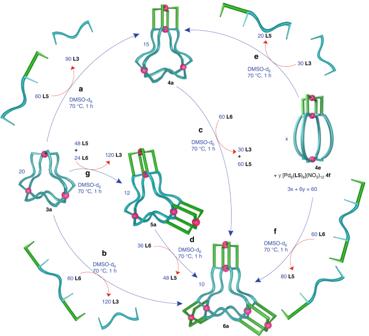Fig. 6: Ligand-displacement-induced cage-to-cage transformations. Initial-cage/ligand-input/final-cage/displaced-ligandasystem3a/L5/4a/L3;bsystem3a/L6/6a/L3;csystem4a/L6/6a/L3&L5;dsystem5a/L6/6a/L5;esystem4e/L3/4a/L5;fsystem4e/L6/6a/L5;gsystem3a/L5&L6/5a/L3(stoichiometry are provided in the figure. The complex4ecoexists with4f). To the solution containing the oligomer, a solution of tetra- n -butylammonium nitrate (0.76 mg, 0.0025 mmol) was added and heated at 70 °C for 20 min resulting the complex [(NO 3 ) 3 ⊂ Pd 6 (L6) 6 ](BF 4 ) 9 , 6a′ . The 1 H NMR spectrum of the complex 6a′ is closely comparable with the data of complex 6a . Complexes [(X) 3 ⊂ Pd 6 (L6) 6 ](BF 4 ) 9 , 6b′−6d′ were prepared in a similar way. (see Supplementary Methods and Supplementary Fig. 94 ).